Observation of decoherence in a carbon nanotube mechanical resonator In physical systems, decoherence can arise from both dissipative and dephasing processes. In mechanical resonators, the driven frequency response measures a combination of both, whereas time-domain techniques such as ringdown measurements can separate the two. Here we report the first observation of the mechanical ringdown of a carbon nanotube mechanical resonator. Comparing the mechanical quality factor obtained from frequency- and time-domain measurements, we find a spectral quality factor four times smaller than that measured in ringdown, demonstrating dephasing-induced decoherence of the nanomechanical motion. This decoherence is seen to arise at high driving amplitudes, pointing to a nonlinear dephasing mechanism. Our results highlight the importance of time-domain techniques for understanding dissipation in nanomechanical resonators, and the relevance of decoherence mechanisms in nanotube mechanics. Decoherence in mechanical resonators corresponds to a loss of phase information of the oscillations in position, similar to decoherence in quantum systems because of the loss of phase information of a superposition state. In contrast, dissipation in a mechanical oscillator or quantum system corresponds to a loss of energy over time [1] , [2] , [3] . The distinction between decoherence and dissipation is often overlooked when studying the quality factor of a mechanical resonator. The mechanical response is typically characterized by a quality factor Q , which is measured from either a spectral response or by a ringdown measurement. In a spectral response measurement, the driving frequency of the resonator is swept and the steady-state oscillation amplitude is measured. From the width of the response peak, a quality factor is extracted. In a ringdown measurement, a quality factor is determined by the envelope of the transient of the resonator after a driving force is switched off. Despite the fact that they are both given the same symbol Q , the quality factors obtained from these two types of measurements are sensitive to different physical processes. The quality factor measured in the spectral response, which we will denote here as Q S , is sensitive to both dissipation (energy loss) and pure dephasing (such as fluctuations of the resonators resonance frequency), similar to the T 2 time in a Ramsey experiment with a qubit [4] . The quality factor Q R measured in a ringdown experiment is sensitive only to dissipation (energy loss), similar to a T 1 measurement on a qubit [5] . In qubits, it is well-known that the T 1 and T 2 can be very different: an extreme example is a GaAs spin qubit, in which T 2 can be as short as 10 ns, whereas T 1 can be as long as 1 s (refs 6 , 7 ). Decoherence in mechanical resonators has been studied earlier in a piezoelectric resonator coupled to a superconducting circuit [8] , in atomically thin drum resonators [9] , and in the two coupled modes of a vibrating string [10] . In these experiments, no pure dephasing was observed and the coherence of the motion was limited by dissipation. In experiments with mass sensing [11] , excess phase noise was observed, which was attributed to surface diffusion of molecules [12] . In comparison to conventional nanoelectromechanical system, carbon nanotube (CNT) resonators are very sensitive to their environment. Owing to a low mass and spring constant, nanotube mechanical resonators show a strong dispersion with the gate voltage [13] , are sensitive to the force of a single-electron charge [14] , [15] , exhibit strong mode coupling [16] , [17] and strong nonlinearities [18] . These strong coupling effects may give rise to dephasing, making them an interesting candidate for exploring mechanical decoherence. Furthermore, the low value of the quality factor in CNT resonators is not well understood. It has been proposed that low Q factors could originate from thermally induced spectral broadening [19] , clamping losses [20] , [21] , [22] or from symmetry breaking [23] . Until now, reports of the quality factor in CNTs have been based only on spectral measurements [14] , [18] , [24] . To distinguish dissipation processes from dephasing, additional measurements, such as a mechanical ringdown, must be performed. Here we use a recently developed fast detection scheme to measure the ringdown of a CNT mechanical resonator [25] . Doing so, we gain access to both the dissipation and decoherence processes. At low driving power, we find that Q S and Q R have the same value, indicating that dephasing processes are not significant. At higher driving power, however, we find that spectral response becomes significantly broader, with a drop in Q S by a factor of four, while Q R remains constant, demonstrating decoherence from dephasing of the nanotube motion. Description and characterization of the device A suspended single-walled CNT mechanical resonator is fabricated as described previously [25] . Briefly ( Supplementary Methods ), fabrication starts with an intrinsic silicon wafer, on which a gate electrode is patterned. On top, a 200-nm-thick silicon oxide layer is deposited, followed by a 70-nm-thick MoRe source and drain electrodes. Finally, a CNT is grown across the 500-nm trench that separates the electrodes. The distance between the gate and the CNT is 270 nm. 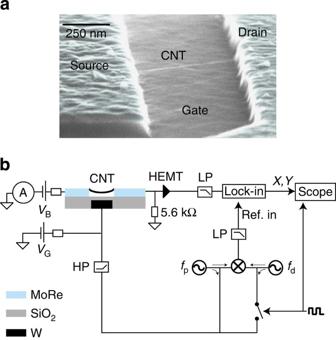Figure 1: Device and measurement setup. (a) Colourized scanning electron microscope image of a typical device, showing a suspended CNT in contact with source and drain electrodes. (b) Schematics of the measurement setup. To measure the mechanical response, two frequency signal generators are used: one for the drive and one for the probe signal. The probe signalfpis detuned by 7 MHz from the drive signalfd. A radio frequency switch is used to turn on and off the drive signal to the gate using square-wave pulses. A mixing signal is generated with a mixer at room temperature, which serves as a reference signal for the lock-in amplifier. A second mixing signal is generated by the CNT, which is impedance-matched by a high electron mobility transistor (HEMT) and detected by a lock-in amplifier. TheXandYquadrature outputs from the lock-in are recorded in sync with the switch by an oscilloscope. In the schematic, HP (LP) represent high (low) pass filters. Figure 1a shows a scanning electron microscope image of a typical device. Figure 1b shows the schematic of the circuit used to measure the conductance of the CNT as a function of gate voltage ( Fig. 2a ). The measurements presented here are performed at 2 K. A high conductance is observed for negative gate voltages, when the CNT is doped with holes. When a positive gate voltage is applied, a low conductance region (small band gap) is followed by weak conductance oscillations because of Coulomb blockade. This overall behaviour is typical for a clean single CNT in contact with MoRe electrodes [26] . Figure 1: Device and measurement setup. ( a ) Colourized scanning electron microscope image of a typical device, showing a suspended CNT in contact with source and drain electrodes. ( b ) Schematics of the measurement setup. To measure the mechanical response, two frequency signal generators are used: one for the drive and one for the probe signal. The probe signal f p is detuned by 7 MHz from the drive signal f d . A radio frequency switch is used to turn on and off the drive signal to the gate using square-wave pulses. A mixing signal is generated with a mixer at room temperature, which serves as a reference signal for the lock-in amplifier. A second mixing signal is generated by the CNT, which is impedance-matched by a high electron mobility transistor (HEMT) and detected by a lock-in amplifier. The X and Y quadrature outputs from the lock-in are recorded in sync with the switch by an oscilloscope. In the schematic, HP (LP) represent high (low) pass filters. 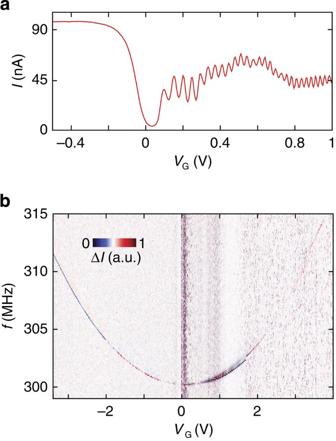Figure 2: Device characterization. (a) Conductance as a function of gate voltageVGat 2 K and atVB=4 mV. ForVG<0 V, the conductance is high, whereas forVG>0 V, the conductance is low, exhibiting weak Coulomb blockade. (b) Resonance frequency as a function of gate voltage, showing that the suspended CNT acts as a gate-tuneable mechanical resonator. Full size image Figure 2: Device characterization. ( a ) Conductance as a function of gate voltage V G at 2 K and at V B =4 mV. For V G <0 V, the conductance is high, whereas for V G >0 V, the conductance is low, exhibiting weak Coulomb blockade. ( b ) Resonance frequency as a function of gate voltage, showing that the suspended CNT acts as a gate-tuneable mechanical resonator. Full size image To find the mechanical resonance and to characterize its gate dependence, we first measure the nanotube motion using the rectification technique outlined in ref. 15 . Figure 2b shows the resonant change in DC current Δ I as a function of frequency f d and V G at V B =1 mV. The frequency at which the mechanical signal is detected increases with gate voltage, characteristic for a CNT mechanical resonator [13] . The approximately quadratic gate voltage dependence suggests that there is some slack in the nanotube. Observation of the mechanical ringdown of a CNT In Fig. 3 , we measure the response of the mechanical resonator in the time domain. The schematic of the detection circuit is shown in Fig. 1b . Two signal generators are used to generate a drive ( f d ) and a probe ( f p ) signal. The amplitude of the drive signal was chosen to be sufficiently small such that mechanical response does not exhibit a nonlinear Duffing line-shape. The probe signal is 7 MHz detuned from the drive frequency and a mixer is used to generate a 7-MHz reference signal for the lock-in. The CNT resonator is driven and detected by applying the drive and probe signals to the gate. The transconductance of the CNT leads to the mixing of these two signals (see Supplementary Notes 1 and 2 and Supplementary Figs 1–3 ). Note that this is slightly different than conventional two-source mixing where one signal is applied to the source and the other to the gate: at cryogenic temperatures, the nonlinear response of the nanotube conductance with gate voltage G ( V G ) allows us to use a similar mixing-type detection [13] with signals applied only to the gate and a constant DC voltage bias V B =−5 mV. To impedance match the signal coming from the nanotube, a high electron mobility transistor (HEMT) is located in close proximity to the CNT, so that the motion can be detected with a bandwidth of 62 MHz (ref. 25 ). Here we use a high-frequency lock-in amplifier to detect the signal from the HEMT amplifier, in which case our readout scheme can detect motion on μ s timescales. 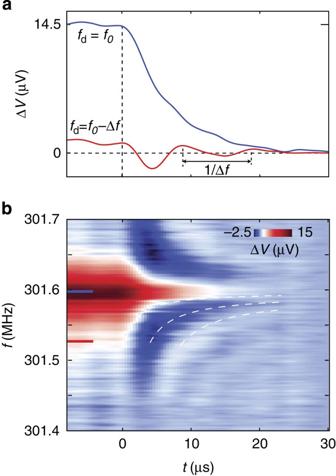Figure 3: Time-domain response of the CNT motion. (a) Recorded response of the lock-in amplifier when switching off the drive signal for an on resonance (blue) and off-resonance (red) drive frequency. The red curve shows the mechanical response of the CNT when the drive signal is detuned by Δf=70 kHz from the mechanical resonance position. An oscillation on top of the ringdown signal (fort>0) is visible. The oscillation periodicity matches with. (b) Colour-scale map of the mechanical ringdown signal as a function of time and drive frequency. A white contour on top of the colour-scale map indicates the peak and dip positions because of the detuning from the fundamental mechanical resonance frequency. The red and blue markers inbindicate the positions where the line-cuts inaare extracted from. Figure 3: Time-domain response of the CNT motion. ( a ) Recorded response of the lock-in amplifier when switching off the drive signal for an on resonance (blue) and off-resonance (red) drive frequency. The red curve shows the mechanical response of the CNT when the drive signal is detuned by Δ f =70 kHz from the mechanical resonance position. An oscillation on top of the ringdown signal (for t >0) is visible. The oscillation periodicity matches with . ( b ) Colour-scale map of the mechanical ringdown signal as a function of time and drive frequency. A white contour on top of the colour-scale map indicates the peak and dip positions because of the detuning from the fundamental mechanical resonance frequency. The red and blue markers in b indicate the positions where the line-cuts in a are extracted from. Full size image To measure the mechanical ringdown, we use the following pulsed excitation and measurement scheme. A switch in the circuit controls the drive signal ( f d ), which is connected to the gate of device. With the switch on, the motion of the CNT is excited. When the switch is turned off, only the probe and an effective gate voltage from the motion of the CNT are present. These two are mixed by the CNT, and the resulting signal is amplified by the HEMT and detected by the lock-in amplifier. The envelope of the mechanical ringdown signal is then detected as a function of time by detecting the output of the lock-in amplifier with an oscilloscope. The blue curve in Fig. 3a shows the transient response measured by the lock-in after the CNT resonator has been driven at resonance ( f d = f 0 ). The gate voltage is fixed at V G =0.4 V and the drive signal is switched off at t =0 μs. To improve the signal-to-noise ratio, the output quadratures from the lock-in have been averaged using the oscilloscope, typically 10,000 times. The averaging was done by applying a repeating square-wave voltage signal to the radiofrequency switch Fig. 1 . The same square-wave signal is used to trigger the oscilloscope. In the data shown, a constant offset from electrical mixing has been subtracted, and the quadratures have been rotated ( Supplementary Note 2 and Supplementary Figs 4–7 ) such that the data presented represent the amplitude of the mechanical signal. The rounding of the decay curve around t =0 is consistent with smoothing on a short timescale from the lock-in filter response (see Supplementary Note 3 and Supplementary Fig. 8 ). The red curve in Fig. 3a shows the response when the drive signal is detuned by Δ f =70 kHz from the mechanical resonance of the CNT [27] . In this case, the signal does not just decay but instead oscillates below the relative zero position, while decreasing in amplitude. This oscillation frequency matches the frequency detuning relative to the mechanical resonance frequency (Δ f = f 0 − f ). The origin of these oscillations lies in the behaviour of a driven mechanical resonator. When driven off-resonance, the motion oscillates at the driving frequency. However, when the driving is switched off, the mechanical resonator oscillates at its natural frequency. Because the reference of the lock-in amplifier is referenced by the initial drive frequency, the output of the lock-in oscillates at the difference frequency Δ f (see Supplementary Note 2 and Supplementary Fig. 7 ). The observation of this oscillation is a clear confirmation that the observed transients are mechanical in nature. To further investigate this behaviour, we plot in Fig. 3b a two-dimensional colour-scale representation of the measured amplitude as a function of time and drive frequency. While keeping the gate voltage V G =0.4 V fixed, we slowly step the drive and probe signal across the mechanical resonance of the CNT. For each frequency, we record the averaged lock-in output quadratures with the oscilloscope. On top of the colour-scale map, a contour map with white dashed lines is shown, to indicate the positions of the peaks and dips of the ringdown signals that are recorded off-resonance. The, dashed lines indicate the expected peak and dip positions with a periodicity of , where Δ f = f 0 − f d is the detuning relative from the mechanical resonance position. As can be seen from the two-dimentional colour map, the dashed lines follow the observed peak/dip positions, confirming that the oscillating ringdown signal is indeed from the mechanical resonator. Decoherence and nonlinear dephasing of the motion of a CNT To extract the ringdown quality factor Q R , we fit the measured time response of device for resonant driving. An important detail in the experiment is that the averaging in the oscilloscope is performed on time traces of the amplitude quadrature. To describe such quadrature-averaged measurements, we introduce a model that includes the effects of dephasing and of the filter response of the lock-in amplifier (see Supplementary Note 3 and Supplementary Figs 8–10 ). This model, which is constrained by the independently observed Q S , allows us to extract Q R from the mechanical transient. In Fig. 4 , we use this technique to independently extract the dephasing and dissipation contributions to the mechanical quality factor. The upper panels show the spectral response and the time-domain response for a low driving power. Fitting the data sets, we find that both Q S and Q R are well described by a single number ( Q S = Q R =6,250) indicating that dephasing does not play a role at this driving power. 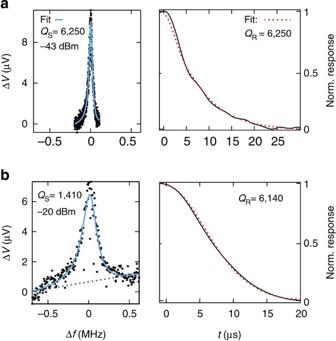Figure 4: Decoherence of a carbon nanotube mechanical resonator. The gate voltageVG=0.4 V and the temperature is 1.9 K. The drive power and fitted quality factor are indicated in the panels. Ina, the probe power is −28 dBm and the resonance positionf0=301.6 MHz. Inb, the probe power is −8 dBm and the resonance positionf0=299.69 MHz. The data were fitted by including a slowly varying frequency-dependent electrical mixing signal (dashed line), seeSupplementary Note 3andSupplementary Figs 9 and 10. We estimate an amplitude of 0.14 and 0.7 nm foraandb, respectively (Supplementary Note 2). Figure 4: Decoherence of a carbon nanotube mechanical resonator. The gate voltage V G =0.4 V and the temperature is 1.9 K. The drive power and fitted quality factor are indicated in the panels. In a , the probe power is −28 dBm and the resonance position f 0 =301.6 MHz. In b , the probe power is −8 dBm and the resonance position f 0 =299.69 MHz. The data were fitted by including a slowly varying frequency-dependent electrical mixing signal (dashed line), see Supplementary Note 3 and Supplementary Figs 9 and 10 . We estimate an amplitude of 0.14 and 0.7 nm for a and b , respectively ( Supplementary Note 2 ). Full size image In the lower panels, we show the mechanical response at higher driving powers. At higher driving powers, the spectral response is still well described by the line-shape of an harmonic oscillator (see Supplementary Note 1 and Supplementary Fig. 1 ) with no sign of hysteresis, indicating that the amplitude of the motion is small enough that nonlinear restoring forces (which would lead to a Duffing response) are not significant. Although the response still fits well to the line-shape of an harmonic oscillator, it has increased in line-width, now exhibiting a Q S =1,410. In the right panels, we show the simultaneously measured time-domain response. Remarkably, although the spectral line-width has increased significantly, the ringdown response decays on a timescale comparable to the data set at a lower power, which showed Q S =6,250. Fitting the data to the model, we find Q R =6,140, a value very similar to that from the lower power data set. Although increasing the drive power significantly increases the spectral line-width, the observed value of Q R shows that dissipation is unchanged. The observation of Q R >> Q S demonstrates the importance of dephasing and decoherence in the dynamics of the CNT motion. We also observe this difference in spectral Q S and ringdown Q R at different gate voltages (see Supplementary Fig. 11 ) In the observations presented here, dephasing appears with increased amplitude of the mechanical motion, indicating a nonlinear dephasing mechanism. We note that a similar observation of an increasing spectral line-width with increased driving power was recently reported as an indication of nonlinear dissipation in graphene resonators at low temperature [18] . Our results here show that such effects in the spectral quality factor Q S can also arise from a power-dependent dephasing mechanism, and that fast time-domain measurements such as those presented here are able to distinguish between the two. Having established the presence of nonlinear dephasing in our device, it is interesting to consider what mechanisms could lead to such an effect. One possible source is an excess voltage noise on our gate: as the mechanical frequency is gate voltage dependent, noise on the gate would give rise to random fluctuations in mechanical frequency, which would increase Q S through spectral (inhomogeneous) broadening. From the dispersion of the mechanical frequency with gate voltage, we estimate that a gate voltage noise of 45 mV would be needed to produce the observed spectral broadening. This corresponds to a gate voltage noise larger than the Coulomb peak spacing (see Supplementary Fig. 12 ). This is significantly higher than the noise level in our setup, suggesting we can rule out gate voltage noise as the origin of the observed effects. Another possibility is effects from the relatively weak Coulomb blockade in our device, in which a fluctuating force from the tunnelling of single electrons could dephase the mechanical motion [28] . Although we did not observe any strong dependence of Q S as the gate voltage was swept across the weak Coulomb blockade features, future experiments at lower temperature where Coulomb blockade effects become more significant could shed light on this mechanism. A third possible source is dephasing from coupling to the stochastic motion of other mechanical modes [19] , [29] , [30] . One way in which mode coupling could explain the amplitude-dependent spectral broadening is through an increased heating of the other modes from the larger driving. These effects could be explored in future experiments through detailed temperature dependence studies. In very recent work [31] , changes in the thermomechanical noise spectrum of a CNT resonator were seen in response to nonlinear driving forces. Such increases in the thermomechanical noise (heating) from large driving amplitudes could also play a role. It is an interesting question if the effects observed in that work could play a role in the spectral- and time-domain mechanical response studied here. In summary, we have used a high-speed readout technique to measure the mechanical ringdown of a CNT. Using this technique, we demonstrate decoherence of the mechanical motion from an amplitude-dependent dephasing process. Future studies of motion in the time domain could potentially identify the origin of this dephasing and explore dissipation and decoherence in CNT motion. How to cite this article: Schneider, B. H. et al . Observation of decoherence in a carbon nanotube mechanical resonator. Nat. Commun. 5:5819 doi: 10.1038/ncomms6819 (2014).